Ubiquitous long-range antiferromagnetic coupling across the interface between superconducting and ferromagnetic oxides The so-called proximity effect is the manifestation, across an interface, of the systematic competition between magnetic order and superconductivity. This phenomenon has been well documented and understood for conventional superconductors coupled with metallic ferromagnets; however it is still less known for oxide materials, where much higher critical temperatures are offered by copper oxide-based superconductors. Here we show that, even in the absence of direct Cu–O–Mn covalent bonding, the interfacial CuO 2 planes of superconducting La 1.85 Sr 0.15 CuO 4 thin films develop weak ferromagnetism associated to the charge transfer of spin-polarised electrons from the La 0.66 Sr 0.33 MnO 3 ferromagnet. Theoretical modelling confirms that this effect is general to all cuprate/manganite heterostructures and the presence of direct bonding only affects the strength of the coupling. The Dzyaloshinskii–Moriya interaction, also at the origin of the weak ferromagnetism of bulk cuprates, propagates the magnetisation from the interface CuO 2 planes into the superconductor, eventually depressing its critical temperature. The interest for superconducting/ferromagnetic (S/F) heterostructures [1] , [2] has been recently renewed by the theoretical predictions of new fascinating interfacial phenomena, such as triplet superconductivity and Π-Josephson effects in mesa-junctions made of two low- T c superconductors coupled through a ferromagnetic barrier [3] . While the understanding of S/F heterostructures based on classical low- T c metals has been progressing considerably [4] , [5] , [6] , a proper description of S/F oxide type interfaces is still lacking, although several intriguing interfacial phenomena have been reported [7] , [8] , [9] , [10] . To date, most work in this field has been focusing on the coupling of YBa 2 Cu 3 O 7-δ (YBCO) and half-metallic manganites, like La 0.66 Ca 0.33 MnO 3 (LCMO) or La 0.66 Sr 0.33 MnO 3 (LSMO), being the superconducting and ferromagnetic layer, respectively. Among these, we cite the ‘induced’ ferromagnetism in the CuO 2 planes [11] accompanied by interface orbital reconstructions [12] , the giant modulation of the magnetisation across the superconducting transition in ferromagnetic manganite layers [13] and the long-range transfer of electron–phonon coupling in oxide superlattices [14] . In YBa 2 Cu 3 O 7 /LCMO superlattices, the weak ferromagnetism in the interfacial CuO 2 planes and the antiferromagnetic (AF) coupling between Cu and Mn spins have both been attributed to the formation of a Mn3 d -O2 p -Cu3 d molecular orbital [14] , [15] . This oxygen-mediated link between copper and manganese ions, perpendicular to the interface, has been assumed to involve only the Cu(2) sites belonging to the superconducting CuO 2 planes, whereas Cu(1) sites, lying in the charge-reservoir and capable of accommodating a variable amount of oxygen by the formation of the so-called chains, are supposed to play no direct role. However, the role of the Mn–O–Cu(2) bridge for the interfacial magnetic coupling, as well as its relationship to the reduced superconducting transition temperatures in cuprate/manganite heterostructures, remains to be demonstrated. In this work, we use atomic layer engineering of complex oxide materials to study the electronic and magnetic properties of cuprate/manganite interfaces characterised by the absence of a direct Cu–O–Mn interfacial bonding. By combining atomic-resolved electron energy-loss spectroscopy (EELS), polarisation-dependent X-ray absorption spectroscopy (XAS) and theoretical modelling, we show that, at the interface with a ferromagnetic manganite, the CuO 2 planes of a superconducting cuprate always develop a weak ferromagnetism, associated with the transfer of the spin-polarised electrons from the bulk of the ferromagnetic metal to the interface. Moreover the magnetisation propagates inside the superconductor via the Dzyaloshinskii–Moriya (DM) interaction and modifies the magnetic correlations within and among the CuO 2 planes, ultimately reducing T c in cuprate/manganite superlattices. Sample fabrication and structural atomic characterisation Superconducting La 1.85 Sr 0.15 CuO 4 (LSCO) ( T c =25 K (ref. 15 )), ferromagnetic LSMO films ( T C =350 K (ref. 16 )) and (LSCO/LSMO) multilayers were deposited by electron diffraction-assisted pulsed laser deposition (PLD) on TiO 2 -terminated SrTiO 3 (001) substrates. The MLs were composed of five stacked (LSMO) m /(LSCO) n bilayer units, with the LSCO thickness fixed at 23 u.c. ( n =23), and the LSMO evolving from m =50 u.c. next to the substrate to m =15 u.c. at the topmost level. In heteroepitaxy both materials grow with their bulk crystalline structure: along the c axis LSMO follows the A O– B O 2 plane sequence of perovskites ( A =La,Sr; B =Mn), while LSCO adopts the A O– C O 2 – A O– A O– C O 2 – A O stacking ( A =La,Sr; C =Cu), where the adjacent A O layers are in-plane shifted. Therefore, two different types of interfaces exist within these heterostructures, depending on the growth sequence (see Fig. 1 ): the first one (type A), with LSCO on top of LSMO, forms a direct Mn–O–Cu bond ( A O– B O 2 – A O– C O 2 – A O); the other (type B), with LSMO deposited onto LSCO, does not have such direct bonding ( A O– C O 2 – A O– A O– B O 2 – A O). The investigation of the type B interface, subject of this contribution, allows clarifying the role of the Mn–O–Cu bridge on the interfacial magnetic coupling by comparing the local magnetic properties through XAS and EELS. 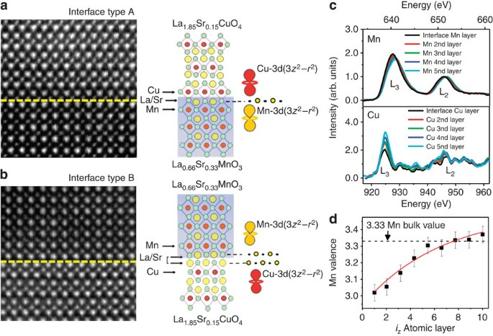Figure 1: STEM/EELS of LSCO/LSMO interfaces with two different atomic stacking sequences. HAADF images of (a) type A and (b) type B interface (left) and the corresponding schematic arrangement of atoms and of Cu and Mn 3dz2orbitals (right). (c) Layer-resolved Mn-L2,3and Cu L2,3EELS spectra; each curve is the average of five spectra acquired sequentially along a lattice plane parallel to the interface (5 pixels of a spectrum image of the near-interface region). A constant background has been subtracted and the spectra have been normalised to the L2edge. The Cu spectra have been smoothed by adjacent averaging. (d) Valence of Mn as function of the atomic layer determined from the O-K spectra of LSMO layer using the method of ref.18which is based on the energy separation ΔEbetween the main peak and the pre-peak as depicted inSupplementary Fig. 3(the red line is a guide for the eye). The error bars are evaluated from the uncertainty in the determination of the relative peak position and from the inaccuracy of the phenomenological relation between ΔEand the actual valence. The error bars are also comparable with the standard deviation of the Mn valence as determined by a statistical analysis over several atomic columns. Figure 1: STEM/EELS of LSCO/LSMO interfaces with two different atomic stacking sequences. HAADF images of ( a ) type A and ( b ) type B interface (left) and the corresponding schematic arrangement of atoms and of Cu and Mn 3 d z 2 orbitals (right). ( c ) Layer-resolved Mn-L 2,3 and Cu L 2,3 EELS spectra; each curve is the average of five spectra acquired sequentially along a lattice plane parallel to the interface (5 pixels of a spectrum image of the near-interface region). A constant background has been subtracted and the spectra have been normalised to the L 2 edge. The Cu spectra have been smoothed by adjacent averaging. ( d ) Valence of Mn as function of the atomic layer determined from the O-K spectra of LSMO layer using the method of ref. 18 which is based on the energy separation Δ E between the main peak and the pre-peak as depicted in Supplementary Fig. 3 (the red line is a guide for the eye). The error bars are evaluated from the uncertainty in the determination of the relative peak position and from the inaccuracy of the phenomenological relation between Δ E and the actual valence. The error bars are also comparable with the standard deviation of the Mn valence as determined by a statistical analysis over several atomic columns. Full size image The exact stacking sequence at the interfaces is illustrated in Fig. 1 by atomically resolved images obtained by scanning transmission electron microscopy (STEM) using a high-angle annular dark field (HAADF) detector. EELS results, with atomic-scale spatial resolution, have been used to determine the chemical species and the oxidation state. In both materials, La(Sr) columns are the brightest and, as Cu is brighter than Mn, the LSCO layers appear overall at lighter grey-tone than LSMO. According to STEM images, at interface A the CuO 2 and MnO 2 planes are separated by one La(Sr)O plane ( Fig. 1a ), and Cu and Mn ions are bridged through an oxygen ion, whereas at interface B two La(Sr)O planes separate the MnO 2 and CuO 2 atomic layers ( Fig. 1b ), and Mn and Cu ions are displaced in the plane by a (1/2, 1/2) vector across the interface. Consequently, interface A is analogous to the Mn–O–Cu bond formed between YBCO and LCMO, whereas the direct Mn–O–Cu bond is absent for interface B. Mapping the Cu and Mn valence across the interface We have mapped the change in the L 2,3 edges of Cu and Mn, and K edge of oxygen across the two interfaces using STEM/EELS. Even in the absence of direct Cu–O–Mn bonding and despite a larger atomic separation, we have observed a substantial charge transfer from the LSMO to the LSCO layer in type B, as shown qualitatively in Fig. 1c , where we plot Mn and Cu L 2,3 EELS spectra across the interface. The spectra show a progressive decrease of Cu and Mn valence, manifested in a change of the L 3 to L 2 ratio, in the layers located at the interface, suggesting a transfer of electrons from the bulk manganite film to the manganite and cuprate interfacial layers [17] , [18] , [19] . To quantify the effect, in Fig. 1d we show the layer-resolved Mn valence calculated from the analysis of O–K-edge spectra [18] , [20] , which is a better quantitative measurement of the Mn-oxidation state ( Supplementary Fig. 3 ) (whereas oxygen K edge spectra can always be used to measure the Mn valence in manganites, it is unrealiable for cuprate superconductors after air exposure. On the other hand, although the Cu L 2,3 spectra are usually too noisy for a quantitative evaluation of the Cu valence, at a qualitative level they undeniably show the progressive increase of electron occupation at the interface). We can see that the Mn valence at the interface is close to Mn 3+ and progressively goes to values slightly above the bulk 3.33 oxidation state expected from the La/Sr ratio. These data indicate that for both MnO 2 and CuO 2 planes the electron occupation is higher at the interface than far from it. Similar results were observed in LCMO/YBCO multilayers [21] , [22] , and it can be interpreted as transfer of electrons from inner manganite unit cells to the interfacial manganite and cuprate layers. Note that the charge transfer takes place over 4–5 layers of both CuO 2 and MnO 2 (that is, 1.6 nm on both sides). Electronic and magnetic properties by X-ray spectroscopy To probe the magnetic properties and the orbital occupation of the interface B, we have used polarisation-dependent XAS at the L 2,3 edges of Cu and Mn, at low temperature (10 K) and in high magnetic field (up to 6 T). In particular we have chosen a multi-layer having, on top of the LSMO/LSCO sequence described above, a thin (6 nm) LSMO film. By recording simultaneously the surface-sensitive (probing depth ~6 nm) total electron yield (TEY) and the bulk-sensitive (probing depth >50 nm) fluorescence yield (FY) signals, we could reliably isolate the signal coming from the shallowest interface, which is of type B ( Supplementary Fig. 5 ). We remind here that by using circularly polarised photons, the X-ray magnetic circular dichroism (XMCD) spectra provide information on the spin and orbital magnetic moments [23] , [24] , [25] , whereas X-ray linear dichroism (XLD) can be used to determine the orientation of the empty 3 d orbitals [26] , [27] . In this way even tiny magnetic moments and orbital anisotropies can be detected. As previously shown in ref. 24 , a small XMCD signal is measured already in isolated LSCO films under a sufficiently strong magnetic field (>1 T), with the sign of the dichroism (negative at L 3 and positive at L 2 in accordance with the usual conventions) proper of a Cu magnetic moment parallel to the applied field. This XMCD signal is due to the canting of the Cu spins out of the CuO 2 planes, it has been found also in other cuprates [24] including YBCO, and it is a consequence of the DM interaction. What happens is that in the strong magnetic field the weak AF coupling between neighbour CuO 2 planes is overcome by the DM interaction, which favours a ferromagnetic alignment of the out-of-plane spin component [24] . On the other hand, at the LSMO/LSCO type B interface, we find a different behaviour. A dichroism signal is observed both at Mn and Cu also in relatively small fields, down to 0.1 T. As shown in Fig. 2 , below 1 T the Cu moments align opposite to the applied field and to Mn spins, but for higher fields the Cu dichroism reverses sign, indicating that above 2 T the Cu and Mn moments are both parallel to the external field. The low-field behaviour is the same as in LCMO/YBCO interface in refs 11 , 28 , 29 , that is, the interfacial CuO 2 planes are antiferromagnetically coupled to the ferromagnetic manganite layers even without a direct Cu–O–Mn bonding and, consequently, without a substantial orbital reconstruction. 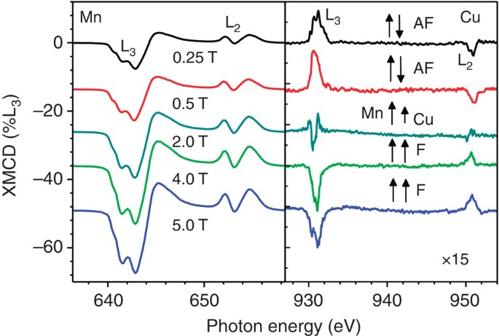Figure 2: XMCD spectra as function of the magnetic field. Evolution vs field of the Mn and Cu L2,3XMCD spectra of a (LSMO)m/(LSCO)23ucmulti-layer covered by a 6 nm ferromagnetic LSMO layer. The spectra, measured by TEY at normal incidence, have been normalised to the maximum of the XAS intensity at L3. The magnetic field was parallel to the incident beam and to the crystallinecaxis. For a more direct comparison, the Cu XMCD signal has been amplified by a factor 15. The AF coupling is compensated by a magnetic field of ~2 T. Figure 2: XMCD spectra as function of the magnetic field. Evolution vs field of the Mn and Cu L 2,3 XMCD spectra of a (LSMO) m /(LSCO) 23uc multi-layer covered by a 6 nm ferromagnetic LSMO layer. The spectra, measured by TEY at normal incidence, have been normalised to the maximum of the XAS intensity at L 3 . The magnetic field was parallel to the incident beam and to the crystalline c axis. For a more direct comparison, the Cu XMCD signal has been amplified by a factor 15. Full size image To identify the role of the orbital occupation on the induced magnetism, we have measured Cu L 2,3 XLD of the interface B. The very-strong linear dichroism, determined by high (very-low) absorption of photons with polarisation perpendicular (parallel) to the c axis, confirms that LSCO at the interface retains the large bulk orbital anisotropy because of the almost exclusive x 2 − y 2 symmetry of the empty 3 d states [26] , [30] . Nonetheless FY and TEY signals show a remarkable difference in the E// c component, as highlighted by the inset of Fig. 3 : after normalisation of the respective in-plane spectra, the TEY spectrum, dominated by the signal from the interface, is two times stronger than the one measured in the bulk-sensitive FY mode. It is also shifted to lower energy, indicating the formation of a state mainly composed by Cu 3 3 d 3 z 2 − r 2 orbitals. However, the redistribution between in-plane and out-of-plane orbitals at the interface is much weaker than reported for LCMO/YBCO SLs [12] . Thus in our LSCO/LSMO multilayers, we observe the same magnetic reconstruction found in LCMO/YBCO, but without substantial modifications of the Cu orbital occupation, as one should expect in the absence of the direct Cu–O–Mn bonding. This means that the AF coupling does not need a straight Mn–O–Cu bridge. 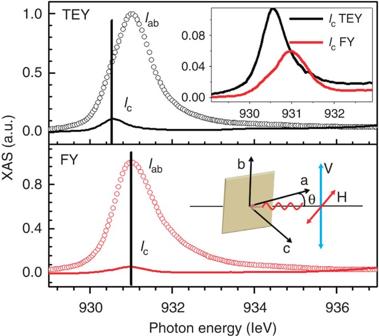Figure 3: Cu L3linear dichroism spectra obtained in TEY and FY configuration. Cu L3XAS, acquired by interface sensitive TEY (top panel) and bulk-sensitive FY (bottom panel);Iab(circles) is the normalised intensity for vertical (V) linear polarisation, parallel to the ab plane;Ic(solid lines) is the corresponding intensity for horizontal (H) polarisation, that is, almost parallel to thecaxis The inset in the top panel shows a direct comparison between TEY (black) and FY (red) with H polarisation. In the bottom panel the experimental setup for XLD is sketched (θ=70°). Figure 3: Cu L 3 linear dichroism spectra obtained in TEY and FY configuration. Cu L 3 XAS, acquired by interface sensitive TEY (top panel) and bulk-sensitive FY (bottom panel); I ab (circles) is the normalised intensity for vertical (V) linear polarisation, parallel to the ab plane; I c (solid lines) is the corresponding intensity for horizontal (H) polarisation, that is, almost parallel to the c axis The inset in the top panel shows a direct comparison between TEY (black) and FY (red) with H polarisation. In the bottom panel the experimental setup for XLD is sketched ( θ =70°). Full size image Theoretical modelling The results are explained quantitatively by a theoretical model capable of reproducing the two following key experimental findings: in both LSMO/LSCO and LCMO/YBCO systems the main electronic modification at the interface with respect to the bulk consists of an increased Cu 3 d 3 z 2 − r 2 character; even in isolated superconducting layers the Cu–Cu DM interaction competes with the weak out-of-plane AF exchange, so that a moderate magnetic field favours a parallel alignment of out-of-plane components of Cu spins even in the bulk ( Supplementary Fig. 6 ), while the in-plane components keep the usual short-range AF coupling. Consequently, by extending the work of Salafranca and Okamoto [31] , we have used a two-band version of cuprate model Hamiltonian, derived from Cu 3 d 3 z 2 − r 2 and 3 d x 2 − y 2 orbitals whose energy separation has been taken from our recent experimental inelastic X-ray scattering studies of ref. 32 ( Supplementary Note 4 and Supplementary Fig. 10 ). For manganites, we consider a single band with e g character ( Supplementary Note 5 ). Compared with the bulk charge distribution, the excess positive charge of the La/Sr layers at the interface B creates an electrostatic potential well. As shown in the Supplementary Notes 6 and 7 and Supplementary Figs 7–9 , these electrostatic effects have been explicitly included in the calculations. The effects of an external magnetic field and two-body interactions, such as DM term in the cuprate, have been included within a low-temperature mean-field approach combining complex magnetic solutions together with superconducting d -wave pairing. Finally, interface effects were simulated by including in the Hamiltonian an explicit tunnelling term for the charge transfer between manganite and cuprate, and a term, called H A , accounting for the inter-layer AF coupling with coupling constant J A [31] . The calculated layer-resolved band occupations indicate that the LSCO and the LSMO electron density profile is perturbed by the combined effect of the potential well and of the charge transfer of spin-polarised electrons from the manganite to the cuprate. As shown in Fig. 4a , the Cu 3 d z 2 orbital is losing electrons at the interface, while remaining essentially unchanged in all the other layers; on the contrary the Cu 3 d x 2 − y 2 electron occupation increases at the interface. These results are confirmed qualitatively by the comparison between orbital selective bulk and interface XAS data ( Supplementary Fig. 5 ). On the other hand the Mn total electron density at the interface is larger than the nominal bulk value 0.66 (in particular it is ~1 at the interface) and decreases to a value close to, but smaller than, the nominal one only after five planes. The theoretical predictions are in fair agreement with the experimental data. The layer-resolved Mn valence measured by EELS of Fig. 1d shows the same trend predicted by theory, with a quite good quantitative agreement. In particular, the interfacial Mn valence evolves from ~3 (electron occupation ~1) at the interface, to ~3.4 (electron occupation ~0.6), slightly larger than the nominal bulk valence, 10 u.c. from the interface. Concerning the electron occupation of copper, a quantitative comparison between experimental results and theoretical calculations is hindered by the low signal-to-noise ratio in the experimental data. Nevertheless we observe a qualitative agreement between the EELS results of Fig. 1c and theory of Fig. 4a , both showing an increase of the interfacial electron occupation. This trend is also confirmed by a comparison between bulk (FY) and interface sensitive (TEY) XAS spectra as shown in Supplementary Fig. 5 . 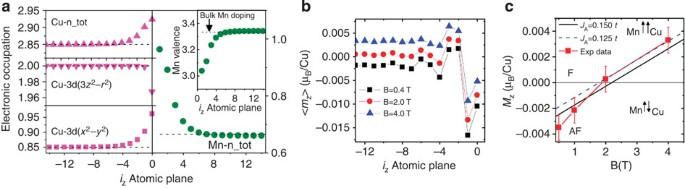Figure 4: Theoretical results of electronic density and magnetisation at the LSCO/LSMO interface, and comparison with experimental results. (a) Calculated 3dorbital occupation for Cu and Mn near the LSCO/LSMO type B interface (seeFig. 1), showing a partial filling of the Cu-dx2−y2states (normally approximately half filled), and a small reduction, at the interfacial CuO2plane only, of the number of electron in the Cu-d3z2−r2states. Similarly, the Mn atoms increase the electronic occupation next to the interface, so that an overall electron-rich region is created across the interface: these electrons are coming from the bulk of LSMO. (b) Calculated magnetisation profile along thecaxis in the cuprate layer in proximity of the interface for different values of the external magnetic field and antiferromagneticJA=0.15t(withthopping integral). (c) Calculated total magnetisation of the cuprate layer as a function of the magnetic field for different values ofJA(black line and dash blue line), compared with the magnetic Cu spin moment determined with sum rules from the experimental XMCD spectra (red square). The error bars for the Cu spin moment indicate the minimum non-zero value detectable in our XMCD experiment. Figure 4: Theoretical results of electronic density and magnetisation at the LSCO/LSMO interface, and comparison with experimental results. ( a ) Calculated 3 d orbital occupation for Cu and Mn near the LSCO/LSMO type B interface (see Fig. 1 ), showing a partial filling of the Cu- d x 2 − y 2 states (normally approximately half filled), and a small reduction, at the interfacial CuO 2 plane only, of the number of electron in the Cu- d 3 z 2 − r 2 states. Similarly, the Mn atoms increase the electronic occupation next to the interface, so that an overall electron-rich region is created across the interface: these electrons are coming from the bulk of LSMO. ( b ) Calculated magnetisation profile along the c axis in the cuprate layer in proximity of the interface for different values of the external magnetic field and antiferromagnetic J A =0.15 t (with t hopping integral). ( c ) Calculated total magnetisation of the cuprate layer as a function of the magnetic field for different values of J A (black line and dash blue line), compared with the magnetic Cu spin moment determined with sum rules from the experimental XMCD spectra (red square). The error bars for the Cu spin moment indicate the minimum non-zero value detectable in our XMCD experiment. Full size image The calculations provide also a layer-resolved map of the Cu spin component along the c axis, that is, perpendicular to the interface ( Supplementary Note 8 ). In a LSCO single layer film, at zero field, the perpendicular component of the magnetisation, related to the spin canting, oscillates around a zero mean value, because of the AF exchange between adjacent CuO 2 planes. On the other hand, the magnetisation profile changes drastically in the case of the cuprate/manganite interface. The first two layers are always antiferromagnetically coupled to the LSMO across the interface ( Fig. 4b ). Thus, the manganite film acts as an exchange biasing field for the weakly ferromagnetic cuprate: below a certain value of the external field (2 T) the antiparallel coupling of the first two Cu layers dominates, so that the overall magnetisation is small with a negative average value and opposite to the manganite ( Fig. 4b ). At higher fields (>2 T), although the antiparallel orientation of the first interfacial planes is maintained, the rest of the LSCO orients parallel to the external field. Indeed, the role of the DM term is to ferromagnetically correlate the out-of-plane component of Cu spins of neighbour CuO 2 planes, while the strong in-plane short-range AF coupling still dominates even at the optimal doping, as demonstrated by the persistence of collective magnetic excitations observed by resonant inelastic X-ray scattering [33] . In Fig. 4c , we show that the calculated average magnetisation along the z axis <m z >=Σ iz m z (iz)/N z is linear as function of the magnetic field for different values of the exchange term J A . It is negative for small magnetic fields, and positive for large fields vanishing at fields of the order of 2 T, in fair agreement with XMCD data (see also Supplementary Figs 11 and 12 ). The comparison with the experimental data (red squares) obtained with the sum rules [23] , [24] , [34] can be used to quantify the value of J A . For LSCO coupled to LSMO (interface B), we have found J A ≈0.15 t , four times smaller than what was estimated in previous experiments for YBCO [31] . The main outcome of this work is schematically pictured in Fig. 5 : the charge transfer of spin-polarised electrons from the manganite to the cuprate layer substantially modifies the magnetisation profile and, eventually, the magnetic correlations of several CuO 2 planes, beyond the interfacial one. It is thus a general property of to cuprate/manganite heterostructures and interfaces. The charge transfer modifies the superconducting doping only within 1–4 CuO 2 layers at the interface while, as shown by our calculations, the magnetisation profile in the cuprate layer is perturbed over at least 10–15 atomic layers, in agreement with the estimates made by Giblin et al. [35] for YBCO/LCMO. The reduction of the critical temperature in our cuprate/manganite multilayers (more than 10 K, see Supplementary Materials ) cannot be explained by the modest change of doping occurring in the first interfacial CuO 2 layers. On the other hand, the perturbation of magnetic correlations among the CuO 2 planes, because of the magnetic proximity effect, extending deeper in the cuprate layers, is likely to have the main role in the suppression of T c . This takes place, for example, by the stabilisation or enhancement of electronic orders in competition with superconductivity (such as the charge ordering recently discovered in the superconducting cuprates [36] ). This interpretation is in agreement with other studies and particular with ref. 8 , where it was demonstrated that the suppression of coherent Drude spectral weight does not take place in SLs where the manganite layer is replaced by a paramagnetic metallic compound like LaNiO 3 , confirming the important role played by the interplay between magnetism and superconductivity in these systems. 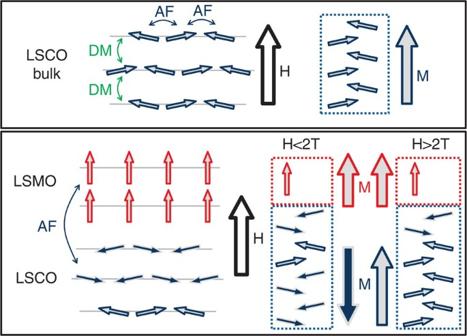Figure 5: Schematic orientation of Mn and Cu magnetic moments across the interface. Top panel: in bulk LSCO a magnetic field H//c induces a net magnetisation because the Cu moments, slightly canted off-plane, couple ferromagnetically their component perpendicular to the CuO2planes under the action of the DM interaction, as previously observed by XMCD24. Bottom panel: at the LMCO/LSMO interface a strong AF coupling between Mn (red/grey) and Cu (blue/grey) moments is established; for relatively weak fields the DM interaction propagates the antiparallel orientation of Cu with respect to Mn far from the interface, whereas for H>2 T the external field establishes a parallel direction as in bulk LSCO. Figure 5: Schematic orientation of Mn and Cu magnetic moments across the interface. Top panel: in bulk LSCO a magnetic field H//c induces a net magnetisation because the Cu moments, slightly canted off-plane, couple ferromagnetically their component perpendicular to the CuO 2 planes under the action of the DM interaction, as previously observed by XMCD [24] . Bottom panel: at the LMCO/LSMO interface a strong AF coupling between Mn (red/grey) and Cu (blue/grey) moments is established; for relatively weak fields the DM interaction propagates the antiparallel orientation of Cu with respect to Mn far from the interface, whereas for H>2 T the external field establishes a parallel direction as in bulk LSCO. Full size image Samples The LSCO/LSMO multilayers, were grown by reflection high-energy electron diffraction-assisted PLD on TiO 2 -terminated SrTiO 3 single crystals, obtained following the Kawasaki technique, in a BHF solution (pH=5.5) [37] , using a KrF laser (λ=248 nm) with fluency of 1.2 J cm −2 and a repetition rate of 4 Hz. During the deposition the temperature was kept at 750 °C in oxygen pressure of 0.2 mbar. After the growth the sample was cooled down in oxygen atmosphere to avoid the formation of oxygen vacancies. The superlattices were characterised ex situ by resistivity and magnetisation measurements ( Supplementary Fig. 1 and Supplementary Note 1 ) with a PPMS (Physical Properties Measurement System) system as function of the temperature. Low-temperature magnetic hysteresis loops on a single LSMO film, showed that the easy axis of magnetisation is parallel to the interface plane, with a coercive field below 0.1 T. By Xx-ray characterisation we found that the c axis of LSCO of 1.32 nm is perfectly correlated to the T c of films deposited by PLD and cooled down in molecular oxygen for the x =0.15 composition, as reported in ref. 28 . STEM and EELS characterisations The structural and chemical integrity of the LSMO/LSCO multilayers were investigated by aberration-corrected STEM and EELS carried out in a Nion UltraSTEM (Nion) microscope operating at 100 keV and equipped with a cold field emission gun, a third generation C 3 /C 5 aberration corrector and a Gatan Enfina EEL spectrometer (Gatan) ( Supplementary Fig. 2 and Supplementary Note 2 ). The abruptness of the interfaces and the interfacial atomic plane stacking were investigated by analysing the normalised integrated intensities of the Cu L 2,3 and the Mn-L 2,3 EELS edges as a function of position, and the intensity of the HAADF images, which is proportional to Z 2 , where Z is the atomic number. Spectrum images were acquired on a 5 × 13 square grid, with spacing equal to ~0.8 a , where a is the pseudocubic LSMO lattice parameter. Within each square, the electron beam performed a subscan on a 16 × 16 grid and the exposure time for each square was set to 2 s. These conditions were chosen to maximize the Cu signal, which tends to be largely masked by the extended fine structure of the strong, preceding La-M 4,5 edge, and to minimize sample drift by reducing the total acquisition time. The spectra were then deconvolved to eliminate the effect of plural scattering through the foil thickness estimated equal to 0.6 λ (λ; electron mean free path) using a low-loss spectrum image collected immediately after the acquisition of the core-loss spectra. XAS, XMCD and XLD measurements Soft XAS was performed at the ID08 beam line of the European Synchrotron Radiation Facility. The APPLE II type undulator source allows a full control of the X-ray beam circular and linear polarisation. The linear polarisation direction, in XLD, could be oriented either in the ab plane of the samples or at an angle from it. Having the polarisation either vertical V or horizontal H in the laboratory frame, with the sample mounted having a vertical ab plane, we measured XAS spectra at the incident angle θ=70° ( Supplementary Note 3 and Supplementary Fig. 4 ). In circular polarisation, we have the XMCD signal, which is the difference in the absorption of light due to a reversal of the light polarisation or magnetisation. The magnetic field can be swept from +5 to −5 T in the direction of the X-rays beam, in a rate of 3 T min −1 . The minimum temperature on the sample is around 8 K. In this experiment up to 32 Cu L-edge XAS spectra, acquired with plus and minus helicities, have been averaged to eliminate any source of systematic error and to reduce the noise level. We have performed measurements in grazing incidence and normal incidence conditions. The sum rules were used to calculate the spin and orbital moments on the Cu L 2,3 edge, following the works in refs 23 , 24 , 34 . During XLD and XMCD experiment the spectra were acquired simultaneously in both FY and TEY configurations. The FY measurements were used to determine the bulk electronic properties (probing a depth of the order of (6–10 nm) of the LSCO superconducting layer ( Supplementary Fig. 5 ). Theory Theoretical calculations are based on inhomogeneous mean-field solutions of the heterostructure. Combined magnetic and superconducting order parameters have been analysed in the cuprate layers. Along the z axis, the size of the cuprate is equal to that manganite and is equivalent to N z =24 planes (see SI-theory). Because of the breaking of the translation invariance along the z axis, order parameters and density occupations are self-consistently calculated plane by plane. How to cite this article: De Luca, G. M. et al. Ubiquitous long-range antiferromagnetic coupling across the interface between superconducting and ferromagnetic oxides. Nat. Commun. 5:5626 doi: 10.1038/ncomms6626 (2014).